Controlling frustrated liquids and solids with an applied field in a kagome Heisenberg antiferromagnet Quantum spin-1/2 kagome Heisenberg antiferromagnet is the representative frustrated system possibly hosting a spin liquid. Clarifying the nature of this elusive topological phase is a key challenge in condensed matter; however, even identifying it still remains unsettled. Here we apply a magnetic field and discover a series of spin-gapped phases appearing at five different fractions of magnetization by means of a grand canonical density matrix renormalization group, an unbiased state-of-the-art numerical technique. The magnetic field dopes magnons and first gives rise to a possible Z 3 spin liquid plateau at 1/9 magnetization. Higher field induces a self-organized super-lattice unit, a six-membered ring of quantum spins, resembling an atomic orbital structure. Putting magnons into this unit one by one yields three quantum solid plateaus. We thus find that the magnetic field could control the transition between various emergent phases by continuously releasing the frustration. It is widely accepted that condensed matter orders at low temperatures by spontaneously breaking some sort of symmetry—translational symmetry in crystalline solids, time reversal and rotational symmetries in magnets, gauge symmetry in superconductors and so on. Whether they can escape from ordering and instead bear emergent states is a question that recurred over decades. A possible strategy to remove trivial orders is to design a model with fine balance of microscopic interactions, where the low-energy states are frustrated and a macroscopic number of quasi-degenerate states compete with each other. When quantum fluctuations between these states prevent a selection of particular order, one ends up with quantum-disordered spin liquids. Modern theories have brought us new insight by identifying spin liquids as topological phases of matter [1] , [2] . Even if such topological phases are not formed, the resultant phase would also be non-trivial; its smallest disentangled unit could consist of several degrees of freedom—pairs of spins in spin ladders or valence bond solids and so on. Thus, characterizing the regime of such liquids and relevant non-trivial phases is now becoming an important challenge. In reality, spin liquids are quite elusive [3] . There are experimental studies on the several materials, suggesting the existence of a spin liquid, κ-(BEDT-TTF) 2 Cu 2 (CN) 3 (ref. 4 ), BaCu 3 V 2 O 8 (OH) 2 (ref. 5 ) and ZnCu 3 (OD) 6 Cl 2 (ref. 6 ). In theories, few candidates include a triangular lattice Mott insulator [7] and spin-1/2 kagome antiferromagnet [8] , [9] , [10] , [11] , represented by the Hubbard and the Heisenberg models, respectively. However, theoretical information directly compared with the experimental data is still severely lacking. Therefore, to find realistic theoretical models that could realize several non-trivial phases and could provide information relevant to experiments is essential. The phase transitions should better be controlled by the experimentally tunable parameter. Here we show that quantum spin-1/2 kagome Heisenberg antiferromagnet in an applied field could be an ideal playground, providing numbers of exotic quantum liquid and solid phases under field control. The model itself is already known as a representative frustrated system that embodies fine balance of interaction by the use of lattice geometry, and, more importantly, it is experimentally relevant. It is defined by the following Hamiltonian: where S i is a spin-1/2 operator at the i -th lattice site ( S i z is the z -component), and J and H are the interaction coupling constant and the external magnetic field, respectively. The first summation denoted by runs over nearest-neighbour pairs of sites of the kagome lattice of size N. The ground state at H= 0 is possibly a spin liquid, but its detailed identification still suffers numerical difficulty. A key numerical problem in quantum many-body models on two-dimensional frustrated lattices is the lack of method that affords sizable results. The quantum Monte-Carlo method suffers from the sign problem, and the exact diagonalization requires unbiased size scaling, which is unavailable at present. Regarding the kagome antiferromagnet, the multiscale entanglement renormalization supported a valence bond crystal ground state with a hexagonal unit cell of 36 spins [11] , which was taken over by a Z 2 gapped spin liquid lower in energy in the latest two-dimensional density matrix renormalization group (DMRG) studies on a long cylinder [8] , [9] . In addition, there is a recent study predicting a gapless U (1) liquid [10] , and the issue remains unsettled. Clarifying the nature of the model in an applied field also demands a severe numerical challenge; the magnetization process appears not as a curve but as a staircase of height ~1/ N owing to finite size effect. Thus, what is known so far is the highly possible presence of a spin-gapped phase called plateau at a 1/3 magnetization [12] , [13] , [14] and a jump of the magnetization from 7/9 to 1 at the saturation field [15] , [16] . Whereas whether a 1/3 plateau is really a plateau [12] , [13] or something else [14] was not really concluded. In the present article, we determine the bulk magnetization process of the kagome Heisenberg antiferromagnet by means of a grand canonical analysis [17] , [18] . The system turns out to have five different plateau phases, and the magnetic field controls the successive phase transitions between these plateau phases and the gapless liquids in a strikingly analogous manner to the Hall conductivity of the quantum Hall effect [19] , [20] , [21] . Two of the plateaus at the lower fields are the possible spin liquids, which are characterized by the finite topological dimensions. The latter three at the higher fields form a long-range order in a particular unit, a hexagonal plaquette consisting of a six-membered ring of spins. This unit resembles a quantum mechanical atomic orbital that accommodates several magnons in its discrete energy levels. The magnetic field thus transforms the system from the highly frustrated liquid phases to the moderately frustrated solid ones. Magnetization curve To overcome the numerical finite size effect, we apply the grand canonical DMRG, which was developed very recently [17] , and was successfully applied to two dimensions [18] . This method gives us a numerically exact and unbiased magnetization curve in the thermodynamic limit (see Methods ). For example, if we choose the cylinder of a finite circumference and of length L , which is larger than ~10–20 lattice spacing, and perform a grand canonical analysis, we obtain a magnetization curve of an infinitely long cylinder of that fixed circumference (see Supplementary Fig. S1 ). As we need a result of a bulk system, equivalently spanned along three different directions of a kagome lattice, we choose a hexagonal cluster for the present calculation rather than a long cylinder. 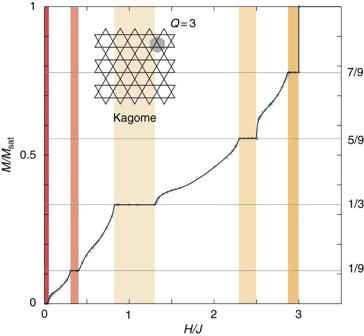Figure 1: Magnetization curve of the spin-1/2 kagome Heisenberg antiferromagnet in a uniform magnetic field. The saturation value of the magnetization density per site isMsat/N=1/2. The inset shows the geometry of the kagome lattice. The shaded hexagon is the original lattice unit cell including three sites (Q=3). Data points are obtained by the grand canonical analysis on a hexagonal cluster withN=114 and 132, which directly gives the curve of the thermodynamic limit without any size scaling. The range of each plateau is highlighted. Figure 1 shows the whole magnetization curve of the kagome antiferromagnet. Without ambiguity, one finds plateau structures at fractions, M/M sat =0, 1/9, 1/3, 5/9 and 7/9, as well as a jump from the 7/9 plateau to the saturation value at exactly H sat /J =3.0, where M sat is the full magnetization. To verify the accuracy of our grand canonical curve, we perform a set of conventional DMRG calculation, both on a long cylinder with open ends (see Supplementary Fig. S1 ) and on an open hexagonal cluster. By comparing these results, we confirm that the grand canonical analysis successfully gives the magnetization curve within the typical accuracy of 10 −3 (see Supplementary Note 1 ). Figure 1: Magnetization curve of the spin-1/2 kagome Heisenberg antiferromagnet in a uniform magnetic field. The saturation value of the magnetization density per site is M sat /N =1/2. The inset shows the geometry of the kagome lattice. The shaded hexagon is the original lattice unit cell including three sites ( Q= 3). Data points are obtained by the grand canonical analysis on a hexagonal cluster with N= 114 and 132, which directly gives the curve of the thermodynamic limit without any size scaling. The range of each plateau is highlighted. Full size image Singlet–triplet spin gap The value of the singlet–triplet spin gap of the kagome antiferromagnet at zero field is still unsettled [8] , [9] , [22] . The evaluated spin gaps after the size scaling in the three latest DMRG studies are not fully consistent; as for the cylindrical DMRG, ref. 9 has Δ =0.13(1) (the numerical data of refs 8 and 9 at various fixed circumferences are basically consistent). There, the size scaling is basically given first along the long leg of a cylinder and the extrapolation is given along the circumference of L ≤20. As for ref. 22 , they increased the size within N =36–108 by keeping the cluster to the square-like shape with periodic boundaries and obtained Δ =0.055±0.005. In fact, we checked these results carefully with the similar scaling and found that the results depend much on the way the size scaling is performed [23] (see Supplementary Notes 1 and 2 ). By contrast, in our grand canonical calculation the size dependence becomes negligible (less than 10 −3 in two dimensions, see Methods ) once we enter a cluster size of the proper system length. Therefore, one could evaluate the spin gap by the onset value of H/J in the magnetization curve near zero field. In Fig. 1 , we find Δ =0.05±0.02 (see the red shaded region), which is obtained on a hexagonal cluster. We briefly mention that our results are fully consistent with the data of the previous conventional DMRG studies: in our grand canonical DMRG on a cylinder with fixed small circumference (see Supplementary Fig. S1 ), the spin gap gives more than twice as large values as the value mentioned above. This value should be compared with the data in ref. 9 on a long cylinder with the same circumference. For a proper extrapolation of the cylindrical results to a bulk two-dimension, one needs to enlarge both the length and the circumferences simultaneously [23] . In fact, our grand canonical spin gap on a hexagonal cluster is very close to those of ref. 22 on a square cluster. Zero and 1/9 plateaus The zero plateau ranging at 0≤ H/J ≤0.05 is the continuation of the zero-field ground state. Correspondingly, in our calculation the spin structure in real space turned out to be completely structureless (see Supplementary Fig. S2 ). One way to identify the nature of the spin liquid is to calculate the von Neumann entropy, S=− Tr( ρ ln ρ ), defined on a subsystem of a long open cylinder by the conventional DMRG, where ρ is the reduced density matrix of the subsystem. The value should follow, S~η L y −γ , where L y is the circumference, η is a constant and γ =ln( D ) is the topological entropy. In ref. 9 , the topological dimension, D , of the ground state is given as D~ 2, which supports the gapped Z 2 spin liquid. In the 1/9-plateau state, the real space profile of the spin structure is rather intriguing, several geometries breaking the translational symmetry are quasi-degenerate (see Supplementary Fig. S2 and Supplementary Note 3 ), and their stability is sensitive to the shape and size of the cluster. We consider this to be the good reason that the symmetry-breaking long order is absent. Therefore, we perform the conventional DMRG and calculate the entanglement entropy of the 1/9-plateau state in the same manner as refs 2 and 9 , as shown in Fig. 2 ; to have the 1/9 magnetization, we need to keep the system size at the multiple of nine, and thus the choice of the clusters are limited compared with the calculation on the M/N= 0 ground state. The topological dimension obtained in the L y =0 limit seemingly gives the value D =3. Thus, the spin-gapped state at 1/9 magnetization is possibly a Z 3 spin liquid, and is the first example of a spin-liquid plateau induced by the magnetic field. Even a Z 3 spin liquid itself has so far been observed only in a specified bosonic model [24] , and the present model gives a more realistic setup. Further examination is required to identify the detailed nature of this phase. 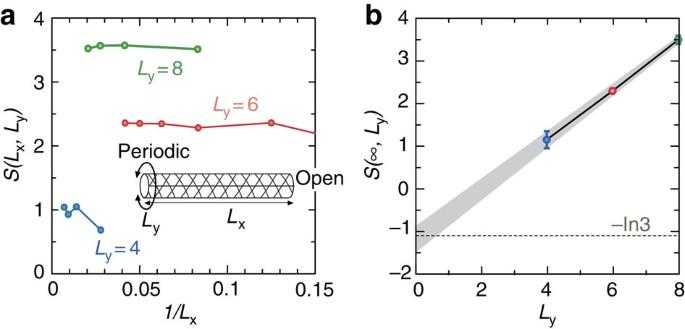Figure 2: Entanglement entropy of a 1/9 magnetization plateau. The results here are calculated on a long cylinder by the conventional DMRG. (a)S(Lx,Ly) as a function of 1/Lxis given forLy=4, 6, 8, whereLxandLydenote the number of sites along the leg and the circumference of the cylinder, respectively. (b) The value extrapolated for the infinite length,Lx=∞, is given as a function of circumferenceLy. The best fit toS=η Ly−γgivesγ=1.18±0.3. We estimate the error in scalingS(Lx,Ly) toLx→∞, which gives the uncertainty of linear scalingS(∞,Ly) againstLy, displayed by grey shading inb. Figure 2: Entanglement entropy of a 1/9 magnetization plateau. The results here are calculated on a long cylinder by the conventional DMRG. ( a ) S ( L x , L y ) as a function of 1/ L x is given for L y =4, 6, 8, where L x and L y denote the number of sites along the leg and the circumference of the cylinder, respectively. ( b ) The value extrapolated for the infinite length, L x =∞, is given as a function of circumference L y . The best fit to S=η L y − γ gives γ =1.18±0.3. We estimate the error in scaling S ( L x , L y ) to L x → ∞, which gives the uncertainty of linear scaling S (∞, L y ) against L y , displayed by grey shading in b . Full size image Long-range ordered plateaus In contrast to the first two plateaus, the rest of the plateaus have symmetry-breaking long-range orders. 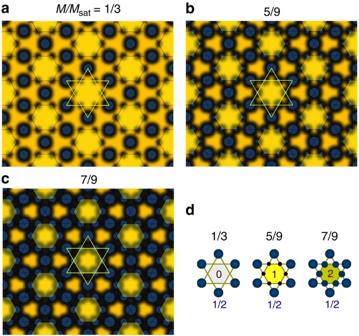Figure 3: Density plot of the magnetization in the long-range-ordered plateau states. The diameter of the blue circle on each lattice site scales the magnetization density. Hexagram consisting of nine sites indicate the magnetic unit cell, extended from the original one by three times (Qmag=9). Hexagons in light yellow colour are the guide to the eye. (d) Schematic alignment of spins on a hexagram, where the numbers indicate the magnetic density (Sz) on each vertices and on hexagons. Numerically, the exact magnetic density of the vertices of hexagram ofaandbare shrunk because of quantum fluctuation by about 2–5% from the fractional values given ind, which is not the case for the 7/9 plateau inc. Figure 3a–c shows the real space profiles of the magnetization density for 1/3, 5/9 and 7/9 plateaus. All of them are based on a same unit of a hexagram, which holds nine lattice sites. This magnetic (extended) unit cell is three times as large as the original unit cell, namely, Q mag =Q × 3=9, with the spin density shown in Fig. 3d . Such symmetry-breaking requires strong interaction between bosons, and the emergence of three such plateaus in a single system is already a quite unexpected matter to happen. Figure 3: Density plot of the magnetization in the long-range-ordered plateau states. The diameter of the blue circle on each lattice site scales the magnetization density. Hexagram consisting of nine sites indicate the magnetic unit cell, extended from the original one by three times ( Q mag =9). Hexagons in light yellow colour are the guide to the eye. ( d ) Schematic alignment of spins on a hexagram, where the numbers indicate the magnetic density ( S z ) on each vertices and on hexagons. Numerically, the exact magnetic density of the vertices of hexagram of a and b are shrunk because of quantum fluctuation by about 2–5% from the fractional values given in d , which is not the case for the 7/9 plateau in c . Full size image In spin-1/2 quantum magnets, a conventional (non-topological) non-magnetic state basically comprises a singlet, a unit of spin 0, often represented by the quantum fluctuation between two spins, (|↑↓ –|↓↑ )/√2. A breaking of singlet yields a bosonic elementary particle carrying spin 1, which is called a magnon. The magnetic field controls the density of these bosons, serving as a chemical potential. As in the Mott insulator, there are particular values of the boson densities commensurate with the lattice periodicity [25] , at which the gapped states are strongly pinned. At these fillings, a finite field range representing the spin gap is formed, which is the magnetization plateau. It is known that the magnetization plateau emerges only when the quantity, Q mag S (1− M/M sat ), is an integer [26] , [27] , where Q mag is the number of sites included in the unit period of the ground state and S is the spin quantum number, which is 1/2 for the present case. With this in mind, let us discuss the nature of our plateaus. We first examine the magnetic structures of M/M sat =0 and 1/9 plateaus, and find that they are possibly structureless in real space (see Supplementary Note 3 ). Namely, the period of the ground state is the same as that of the lattice unit cell, Q mag = Q =3, which gives, Q mag S (1− M/M sat )=3/2 and 4/3, respectively. As they are not integers but fractional numbers, the above conventional condition to have a plateau is not fulfilled. However, in two dimensions there is another way to form a spin-gapped state (plateau) other than the above mentioned interplay with the lattice; it is to form a structureless spin liquid. The elementary excitation of such spin liquids by the magnetic field is no longer a magnon, but a deconfined spinon, carrying spin 1/2. Although such exotic spin-liquid plateaus could emerge at a fractional value of Q mag S (1− M/M sat ), as discussed in field theoretical study [28] , it had been observed neither in theoretical models nor in materials. In fact, the calculations on the entanglement entropy indicate that zero-th and the 1/9 plateau form the spin-liquid phases of topological dimension D= 2 and 3, respectively. In contrast, in the latter three plateaus we find Q mag S (1− M/M sat )=3, 2 and 1 (integers) for 1/3, 5/9 and 7/9 plateaus, respectively, all of which clearly fulfill the above conventional condition. Let us now discuss the origin of these solid plateaus. In the 1/3 plateau, each triangular unit should hold a net magnetization of 1/2, which consists of one up spin 1/2 and two spins forming a singlet (see Fig. 4a ). Similar to the zero-field Ising ground state, there are massive numbers of configuration of the 1/2-magnetized triangular units [29] , which is in fact a typical characteristic of the frustrated system. If these configurations are mixed-up quantum mechanically, a liquid phase should emerge. To realize instead the solid state actually observed, one needs to select a particular configuration, and the problem reduces to how we pave this triangular unit on the kagome lattice to maximally gain energy. 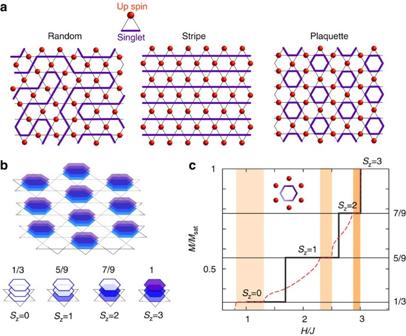Figure 4: Details of the effective model describing the upper three plateau states. (a) A unit triangle at 1/3 plateau includes one up spin (red circle) and two spins forming singlet bond (blue bond). The left panel gives one snapshot of random configuration of unit triangles, which includes winding singlet loops of several lengths. Other two panels are the regular configurations in which the singlet bonds form stripes and hexagonal plaquettes. The latter plaquette long-range order is formed in the 1/3 plateau. (b) Schematic illustration of the three energy levels in each hexagonal plaquette unit. By putting in magnons from the empty level at 1/3 plateau, the 5/9, 7/9 and the fully polarized states are formed. (c) Solid line is the magnetization step of the isolated hexagon in an effective field,H+Hint, whereHint=−Jis from the surrounding six vertex sites indicated in red circles. Broken line is the bulk magnetization curve ofFig. 1. SeeSupplementary Fig. S3andSupplementary Note 4for more details. Figure 4: Details of the effective model describing the upper three plateau states. ( a ) A unit triangle at 1/3 plateau includes one up spin (red circle) and two spins forming singlet bond (blue bond). The left panel gives one snapshot of random configuration of unit triangles, which includes winding singlet loops of several lengths. Other two panels are the regular configurations in which the singlet bonds form stripes and hexagonal plaquettes. The latter plaquette long-range order is formed in the 1/3 plateau. ( b ) Schematic illustration of the three energy levels in each hexagonal plaquette unit. By putting in magnons from the empty level at 1/3 plateau, the 5/9, 7/9 and the fully polarized states are formed. ( c ) Solid line is the magnetization step of the isolated hexagon in an effective field, H + H int , where H int = −J is from the surrounding six vertex sites indicated in red circles. Broken line is the bulk magnetization curve of Fig. 1 . See Supplementary Fig. S3 and Supplementary Note 4 for more details. Full size image In each configuration, one could draw a string along the singlet bonds of the triangular units as shown in the left panel of Fig. 4a . As every triangle shares its corners with the neighbouring triangles, the string never crosses with other strings, but continues until it meets itself again (otherwise it will extend toward infinity). In addition to the random configuration of strings, the representative two regular patterns are shown in Fig. 4a : a long string forming stripes and a shortest closed loop around the hexagon. One then needs to know which gains the energy, the longer string or the shorter loop, towing to the quantum mechanical resonance of spins along the string. The answer is the latter (see Supplementary Fig. S3a )—the kagome is fully tiled with hexagrams—a symmetry-breaking plaquette order is formed [30] . Once all the vertices of the hexagram (three sites/nine unit) are filled with a fully polarized up-spin moment ( S z =1/2) at M/M sat =1/3, a further simplified picture may work, focusing on each hexagonal plaquette and isolating it by effectively neglecting the quantum fluctuation between the plaquette and the vertices of the hexagram, as shown in Fig. 4b . This approximation is valid as far as the vertices of the hexagram are fully polarized. The interactions ( J S z S z -term) between the plaquette and vertices work as an internal magnetic field, H int =− J per site on a plaquette. Figure 4c shows the magnetization process of the isolated plaquette in an effective field, H+H int , namely the doping of magnons by the effective chemical potential. Each step of the big staircases corresponds to the increasing S z -value or the number of magnons in the isolated plaquette. Now, notice that the point where the upshift of the staircases crosses the bulk magnetization curve coincides with the inflection point of the curve. This indicates the following scenario: if we condense the massive numbers of hexagrams, the quantum fluctuations between them become coherent throughout the system and works to destroy the staircases from the edge toward the centre of the step. The curve above/below the inflection point is the ruin of the edge of upper/lower staircase. This result thus supports the picture that a hexagon works as a self-organized pseudo atomic orbital consisting of three discrete energy levels. Doping magnons to each level yields a series of plateaus starting from 1/3. At present, the only other quantum magnet that possibly reveals comparably rich phase transitions is the SrCu 2 (BO 3 ) 2 (refs 31 , 32 ). However, the spin-gapped phases of this material are based on a conventional singlet. In forming solids, they expand the unit cell in several ways to allocate the singlets in a regular period in a sea of doped magnons. In contrast, in our kagome a single non-trivial unit based on a hexagram is self-organized by the quantum many-body effect. The doped magnons come into this cell in such a way that the electrons go into the quantum dots in an artificial semiconductor device. The above picture then gives a strategy to design a system that could control the degree of frustration by the doping of particles; First, prepare an unfrustrated unit that could store several numbers of particles (in a kagome, this corresponds to a hexagon that could hold three magnons). Then connect them by the frustrated bonds. For example, this rule gives us a checkerboard lattice and its relevant pyroclore lattice. Their undoped ground states could be a spin liquid as far as the microscopic interactions are finely balanced. We predict that dopings will also give rise to interesting states of matter similar to the one we find in the kagome. We further pay attention to the fact that the bose-Hubbard model at zero field [33] and the projected quantum dimer model [34] , both on the same kagome lattice, are considered to have Z 2 liquids. Then, one may also expect the 5/9 and 7/9 plateaus to undergo a solid-to-spin-liquid transition [28] if the additional effect enhancing the quantum fluctuation is added to the Hamiltonian. The present findings will give some clue to find numbers of such exotic state of matter in kagome and in the above mentioned lattice models, many of which are still unexplored. Regarding the laboratory systems of the kagome Heisenberg antiferromagnet, there are several candidates, for example, BaCu 3 V 2 O 8 (OH) 2 (ref. 5 ), ZnCu 3 (OH) 6 Cl 2 (ref. 6 ), Cu 3 V 2 O 7 (OH) 2 ·2H 2 O (ref. 35 ) and Rb 2 Cu 3 SnF 12 (ref. 36 ), whereas they are often distorted, anisotropic or include complicated interactions, and the establishing of the ideal kagome Heisenberg material is long awaited. Our bulk magnetization curve is the only data numerically obtained in lattice models that could be compared directly and quantitatively with experimental measurements. Such comparison could be used to identify them as an ideal kagome. Also, if a 1/9 plateau were to appear in the experimental magnetization curve, one could examine, by neutron measurements or some other local magnetic probe-like nuclear magnetic resonance, whether the state is structureless in reality. The magnetic-specific heat and thermal conductivity measurements could further give theorists a hint to know what kind of non-magnetic and magnetic elementary excitations are possible for this newly emergent phase. Thus, our present findings would provide, both in theories and in experiments, a rich playground in search of open paradigms in quantum many-body physics. Grand canonical analysis The technique is developed very recently by the authors [17] , [18] , and gives the infinitesimally small response to the change in the external field. The physical quantities we get mimic their thermodynamic limit within the order of 10 −4 for one dimension and 10 −3 for two dimensions, even in a relatively small cluster size of the order of N~ 10–100. We briefly summarize the essential framework; the method smoothly divides the finite size cluster into the centre part and the edges, and the main part reproduces the continuous bulk response by using the nearly zero-energy edge state as a buffer. At a fixed system size and shape, we introduce the modulation of the energy scale by an externally given function, f( r ), at a location r , which smoothly deforms the Hamiltonian from the maximum at the centre of the system ( r =0) to zero energy at the open cluster edges ( r=R ). After we obtain the proper eigen wave function of the deformed Hamiltonian, we evaluate the magnetization, . Now, remind that the total magnetization, , of the deformed Hamiltonian is a conserved quantity given by hand. However, the expectation value of the local magnetic density is no longer equal to M g /N , but has a particular r -dependence: it takes nearly a uniform value at the centre (though oscillating slightly, the mean values are uniform) and then often takes a peak or valley at the edges (see Suppplementary Fig. S4b and Suppplementary Note 5 ). This is because the system optimizes the wave function so as to realize the centre value, S z ( r ~0) , to its thermodynamic limit, M/N , at a given magnetic field. The excess/deficient magnetization, M g −M , is absorbed/provided by the localized edge states of the cluster, which has the measure zero energy as f( r =R) ~0. These edges serve as a grand canonical bath. The cluster and the function used in the present calculation are given in Supplementary Fig. S4a . The numerical solver of the deformed Hamiltonian is not necessarily restricted to DMRG. The reason why such mechanism works is discussed in detail in ref. 18 in the context of real space energy renormalization, together with applications to several two-dimensional quantum spin systems and to the electronic systems. Details of the DMRG calculation We have used the DMRG [37] as a solver of the deformed Hamiltonian of the ground canonical analysis. The accuracy of the results is systematically controlled by the number of basis states kept, m in the DMRG calculation and the typical error in the energy of the present calculations is around 10 −4 for m= 4,000. As discussed in the Results section, the aspect ratio closer to 1 gives the results closer to the bulk limit. Therefore, we adopt the hexagonal cluster of N =114 and 132, instead of a long cylinder. More details, including the numerical details of the results, are available in the Supplementary Fig. S4 and Supplementary Note 5 . Regarding the calculation on the entanglement entropy in Fig. 2 , we used the conventional DMRG on a long cylinder with open edges and periodic circumferences. There, the number of states kept are m =2,000–10,000, and the data points displayed in Fig. 2a are derived after the extrapolation to 1/m =0. How to cite this article: Nishimoto, S. et al . Controlling frustrated liquids and solids with an applied field in a kagome Heisenberg antiferromagnet. Nat. Commun. 4:2287 doi: 10.1038/ncomms3287 (2013).